Electrically driven polarized single-photon emission from an InGaN quantum dot in a GaN nanowire Since the early demonstration of a quantum dot (QD) single-photon source [1] , [2] , [3] , [4] , [5] , there have been numerous reports on single-photon emission in a wide range of temperatures, with or without the use of a microcavity and with optical or electrical excitation [1] , [2] , [3] , [4] , [5] , [6] , [7] , [8] , [9] , [10] , [11] , [12] , [13] , [14] , [15] , [16] , [17] , [18] , [19] , [20] . Generally, the electrically driven single-photon emitters are all-epitaxial heterostructures. However, polarization control is not easily achieved. For quantum cryptography protocols based on polarization encoding, it is desirable to have a single-photon source whose output is not randomly polarized, but has a fixed polarization depending on the size and shape of the emitter [21] , [22] . GaN and In(Ga)N nanowires can be epitaxially grown catalyst free on silicon substrates with aerial density in the range of 10 8 –10 11 cm −2 and lengths up to a few micrometres [23] , [24] , [25] , [26] , [27] , [28] , [29] , [30] , [31] , [32] . The nanowires grow vertically in the wurtzite crystalline form and optical emission from them in the spectral range of 366–700 nm has been recorded by varying the In composition. Extensive structural characterization indicates that the nanowires are relatively free of extended defects [23] , [24] , [27] , [28] , [29] , [31] , [32] , [33] , [34] . They can be doped p- and n-type with suitable dopant species up to levels similar to those achieved in planar structures. The surface recombination velocity in GaN nanowires is ~10 3 cm s −1 , two orders of magnitude smaller than that on a planar surface of GaAs (ref. 35 ). It is possible to grow one or multiple In(Ga)N disks in Al(Ga)N nanowires to provide quantum confinement, such as in a quantum well [36] , [37] , [38] . However, due to the radial strain relaxation during growth, the piezoelectric polarization field in the disks can be much smaller than in equivalent quantum wells. If the diameter of the nanowire is made small enough and the thickness of the disk is ~2-3 nm, then quasi-three-dimensional confinement, or a QD, is realized. In this bottom-up growth approach, the size of the nanowire and therefore the size of the QD can be carefully controlled. In this work we have investigated single-photon emission from a single In 0.25 Ga 0.75 N QD in a single GaN nanowire with electrical injection. The GaN nanowire contains a p–n junction, and the injected electrons and holes recombine in the In 0.25 Ga 0.75 N QD. The InGaN/GaN dot-in-nanowire heterostructure was grown by plasma-assisted molecular beam epitaxy (PA-MBE) on silicon. The single dot/nanowire junction diode is fabricated on (001) silicon and the experiments have been performed at an ambient temperature of 10 K. The junction temperature is estimated to be higher due to Joule heating, as discussed later. Sharp exciton and biexciton transitions are observed at λ =436.56 nm and 435.03 nm, respectively, in the electroluminescence spectra. Single-photon emission is observed at the biexciton emission wavelength with a value of the second-order correlation function g (2) (0) equal to 0.25. The emitted photons are linearly polarized along the c axis of the nanowire. The radiative lifetime of biexciton emission obtained from time-resolved photoluminescence (TRPL) measurements is 711 ps, and this value is in excellent agreement with the value of the lifetime obtained from analysis of second-order correlation data. Single-photon emission with a larger recombination lifetime of 1.1 ns was also observed at the exciton energy. The value of g (2) (0) for the exciton transition is 0.16. Epitaxial growth and structural characterization The device used to demonstrate single-photon emission in this work was a GaN nanowire p–n junction with an InGaN dot in the active region. The InGaN/GaN dot-in-nanowire heterostructure, shown schematically in Fig. 1a for a single nanowire, was grown on (111) Si substrate by PA-MBE. Catalyst-free growth of the nanowire sample was carried out under nitrogen-rich conditions (see Methods ). Each individual nanowire contains a single InGaN QD, surrounded by undoped GaN barriers, grown on top of Si-doped GaN (n-GaN). At this stage, the nanowire (and QD) diameter is ~25 nm. Following the growth of the QD and GaN barrier, Mg-doped GaN (p-GaN) was grown on top at a lower substrate temperature. The grown sample was structurally characterized by scanning electron microscope (SEM) imaging, seen in Fig. 1b , which yields a nanowire density of ~10 11 cm −2 . 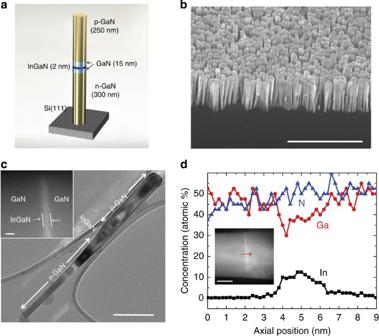Figure 1: Structural characterization of InGaN dot-in-nanowire p–n junction. (a) Schematic of an InGaN dot-in-GaN nanowire p–n junction grown on (111) silicon by molecular beam epitaxy. The 2-nm quantum dot is placed at the centre of doped GaN regions. (b) Scanning electron micrograph of the cleaved edge of an as-grown nanowire sample imaged at a tilt of 45°. The nanowire density is ~1011cm−2. The scale bar denotes 1 μm. (c) Transmission electron micrograph of a single nanowire. The scale bar denotes 100 nm. The lower growth temperature during p-GaN growth leads to an increase in lateral growth rate, and consequently the nanowire diameter increases. The diameter near the centre of the nanowire p–n junction, where the quantum dot is located, is 25 nm. The inset shows a high-resolution image of the In0.25Ga0.75N quantum dot region. The scale bar in the inset is 2 nm. (d) EDX measurement showing the axial profile of elemental composition. Inset shows high-angle annular dark field image of the GaN/In0.25Ga0.75N/GaN heterostructure. The arrow indicates the path of the EDX line scan. The width of the In peak is 2-nm full-width at half maxima. Scale bar: 10 nm. Figure 1c shows the transmission electron microscope (TEM) image of a single nanowire diode. The structure of the InGaN QD was studied by scanning TEM (STEM). As seen in the high-resolution image in the inset of Fig. 1c , both InGaN and GaN regions have perfect crystalline structure. The InGaN/GaN interface appears to be smooth and free of stacking faults. STEM imaging performed on several single dot-in-nanowire samples reveals that the QD diameter and thickness are 25±5 nm and ~2 nm, respectively. Energy-dispersive X-ray (EDX) spectroscopy was performed to confirm the location, composition and thickness of the QD region. An EDX line scan with a 0.2-nm resolution was performed along the nanowire growth c axis (indicated by the arrow) and the results are shown in Fig. 1d . An average alloy composition of In 0.25 Ga 0.75 N in the QD is derived. Additionally, we have grown InGaN nanowires of the same composition as the InGaN dots in the experimental samples and under identical growth conditions. EDX measurements performed on the nanowire ensemble yield an alloy composition of In 0.23 Ga 0.77 N, confirming the result of the EDX measurement on the single dot-in-nanowire (see Supplementary Fig. S1 ). Figure 1: Structural characterization of InGaN dot-in-nanowire p–n junction. ( a ) Schematic of an InGaN dot-in-GaN nanowire p–n junction grown on (111) silicon by molecular beam epitaxy. The 2-nm quantum dot is placed at the centre of doped GaN regions. ( b ) Scanning electron micrograph of the cleaved edge of an as-grown nanowire sample imaged at a tilt of 45°. The nanowire density is ~10 11 cm −2 . The scale bar denotes 1 μm. ( c ) Transmission electron micrograph of a single nanowire. The scale bar denotes 100 nm. The lower growth temperature during p-GaN growth leads to an increase in lateral growth rate, and consequently the nanowire diameter increases. The diameter near the centre of the nanowire p–n junction, where the quantum dot is located, is 25 nm. The inset shows a high-resolution image of the In 0.25 Ga 0.75 N quantum dot region. The scale bar in the inset is 2 nm. ( d ) EDX measurement showing the axial profile of elemental composition. Inset shows high-angle annular dark field image of the GaN/In 0.25 Ga 0.75 N/GaN heterostructure. The arrow indicates the path of the EDX line scan. The width of the In peak is 2-nm full-width at half maxima. Scale bar: 10 nm. Full size image PL and electroluminescence measurements Temperature-dependent PL spectra from an identical QD-nanowire ensemble sample, without the p-GaN grown on top, are presented in Fig. 2a . Strong InGaN QD emission was observed at a wavelength of ~450 nm, with a linewidth of ~14 nm, which is similar to that reported for planar InGaN/GaN single quantum wells [39] . As nanowires are non-resonantly excited, weak emission from GaN is also seen at ~358 nm. The blue shift of the GaN emission compared with the 365-nm emission of bulk GaN is a signature of quantum confinement in the nanowires [40] . The temperature variation of the InGaN QD luminescence peak is plotted in Fig. 2b and the trend is analysed with the Varshni equation [41] . The S-type behaviour is not seen, indicating the absence of any significant compositional inhomogeneity or clustering in the InGaN region [42] , [43] , [44] . A radiative efficiency η r of 52% is estimated from the temperature-dependent data, assuming that the non-radiative recombination centres are frozen at 10 K (see Supplementary Fig. S2 ). 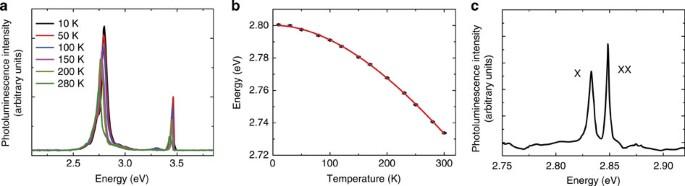Figure 2: InGaN quantum dot photoluminescence. (a) Temperature-dependent photoluminescence spectra from the as-grown nanowire ensemble shown inFig. 1b. The integrated intensity of the quantum dot emission at room temperature is about half of that at 10 K. (b) Peak energy of quantum dot emission fromFig. 2aplotted as a function of temperature with error bars representing the uncertainty due to the finite resolution of the measurement system. The solid line is the calculated variation using the Varshni equation. The Varshni parameters used for the fit areα=(8.3±0.4) × 10−4eV K−1andβ=825±16.7 K. (c) Micro-photoluminescence from a single In0.25Ga0.75N/GaN QD in nanowire at 10 K, obtained from a sample with dispersed nanowires. The excitation power was 400 μW. Figure 2: InGaN quantum dot photoluminescence. ( a ) Temperature-dependent photoluminescence spectra from the as-grown nanowire ensemble shown in Fig. 1b . The integrated intensity of the quantum dot emission at room temperature is about half of that at 10 K. ( b ) Peak energy of quantum dot emission from Fig. 2a plotted as a function of temperature with error bars representing the uncertainty due to the finite resolution of the measurement system. The solid line is the calculated variation using the Varshni equation. The Varshni parameters used for the fit are α =(8.3±0.4) × 10 −4 eV K −1 and β =825±16.7 K. ( c ) Micro-photoluminescence from a single In 0.25 Ga 0.75 N/GaN QD in nanowire at 10 K, obtained from a sample with dispersed nanowires. The excitation power was 400 μW. Full size image Nanowires with p–n junctions were removed from the as-grown substrate and transferred to an oxide-coated silicon wafer, to artificially obtain a nanowire density of ~10 8 cm −2 . Single nanowires chosen after SEM imaging were contacted using electron beam lithography and electron beam evaporation techniques (see Methods ). Micro-PL from a single dot-in-nanowire measured at 10 K, seen in Fig. 2c , exhibits sharp transitions in the blue spectral range, originating from the InGaN QD. Excitation power-dependent measurements confirm these peaks originate from the exciton and biexciton transitions. Measured room temperature current–voltage characteristics of the single QD-nanowire p–n junction (seen in Fig. 3a ) are presented in Fig. 3b . The series resistance of the diode was carefully measured at room temperature (see Supplementary Fig. S3 ) and a value of 2.38 GΩ is derived in the bias range of 2–20 V, in which single-photon measurements have been made. The diode has a very small reverse current (~1 pA) and exhibits no breakdown up to a reverse bias of 20 V. We have measured several single nanowire p–n junction diodes and their characteristics are similar. Typical electroluminescence (EL) spectra from the nanowire-QD device under forward bias at different injection currents are shown in Fig. 3c . Sharp resonances with linewidths ranging from 2 to 3 meV are observed in the spectra. At low injection currents, a sharp peak at 2.84 eV is observed. The integrated intensity of the peak increases linearly with the injection current ( I 1.04±0.02 ). With increase in injection current, a second peak is observed at ~2.85 eV, which increases quadratically with injection current ( I 1.93±0.09 ). The linear and quadratic dependence of intensity on injected current and their subsequent saturation, as seen in Fig. 3d , confirm that the resonances are from single exciton and biexciton transitions, respectively. The measured negative biexciton binding energy of 10 meV is in the range of previously reported values for single InGaN QDs [45] . 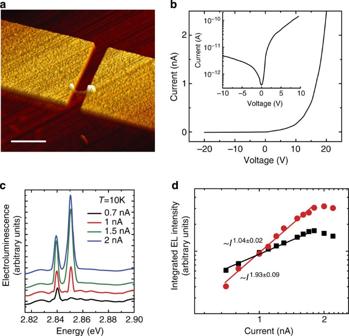Figure 3: Electroluminescence from InGaN dot-in-nanowire p–n junction diode. (a) Atomic force microscope image of a single dot-in-nanowire diode on (001) Si with Ti/Au ohmic contacts. The scale bar denotes 1 μm. The total thickness of the contacts is 50 nm. (b) Room temperature current–voltage characteristics measured after annealing the contacts at 450 °C in N2. (c) Electroluminescence from the dot-in-nanowire diode measured at 10 K for injection currents varying in the range 0.7–2.5 nA. (d) Integrated electroluminescence intensity of the exciton (squares) and biexciton (circles) transitions plotted as a function of injection current obtained from the data ofc. The calculated solid lines indicate that the intensity of the exciton transition increases linearly with injection current (I1.04±0.02) and that of the biexciton transition increases quadratically with injection current (I1.93±0.09). Figure 3: Electroluminescence from InGaN dot-in-nanowire p–n junction diode. ( a ) Atomic force microscope image of a single dot-in-nanowire diode on (001) Si with Ti/Au ohmic contacts. The scale bar denotes 1 μm. The total thickness of the contacts is 50 nm. ( b ) Room temperature current–voltage characteristics measured after annealing the contacts at 450 °C in N 2 . ( c ) Electroluminescence from the dot-in-nanowire diode measured at 10 K for injection currents varying in the range 0.7–2.5 nA. ( d ) Integrated electroluminescence intensity of the exciton (squares) and biexciton (circles) transitions plotted as a function of injection current obtained from the data of c . The calculated solid lines indicate that the intensity of the exciton transition increases linearly with injection current ( I 1.04±0.02 ) and that of the biexciton transition increases quadratically with injection current ( I 1.93±0.09 ). Full size image It is important to note at this point that because of Joule heating caused by the large series resistance of the nanowire diode, the real device (and hence the InGaN QD) temperature might be significantly larger than the ambient temperature of 10 K. We have performed a simulation of the heat-transfer problem by solving the Laplace equation (see Methods ). 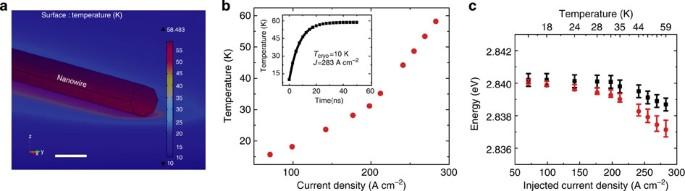Figure 4: Single dot-in-nanowire p–n junction diode temperature. (a) Steady-state spatial temperature profile of a 600-nm-long nanowire of 30 nm diameter placed on a Si/SiO2platform for an injection current density of 283 A cm−2. The scale bar denotes 30 nm. The silicon substrate is maintained at 10 K and the final nanowire temperature is ~59 K. (b) Calculated device temperature for different values of current density. The inset shows the transient response of the nanowire temperature for an injected current density of 283 A cm−2. The transient response depends on the thermal resistance and capacitance of the system. (c) Emission energy shift as a function of the injected current density. The dots represent energy values calculated with the Varshni equation for equivalent temperatures corresponding to the current densities, obtained from the data shown inb. The error bars represent uncertainties in the Varshni fitting parameters. The squares represent measured variation of the exciton emission peak energy with injection current. Errors in the measurement arise from the resolution of the monochromator. Figure 4a shows the simulated nanowire temperature distribution at steady state at a current density of 283 A cm −2 ( I =2 nA). While the generated heat is effectively dissipated by silicon through SiO 2 , the finite heat conductivity of SiO 2 results in a steady-state temperature as high as 60 K in the nanowire. The junction temperature was similarly simulated for other injection currents at an ambient temperature of 10 K and the results are shown in Fig. 4b . As the injection current increases, the calculated steady-state temperature increases quadratically as the heat generation is proportional to the square of the current. As shown in the transient profile in the inset of Fig. 4b , the temperature of the device reaches steady state within 30 ns. Hence, in electroluminescence measurements, any transient temperature effect can be ignored and the injected currents determine the device temperature. In Fig. 4c , we plot the ideal variation of the In 0.25 Ga 0.75 N emission peak with current density, calculated from Varshni coefficients that were previously derived ( Fig. 2b ) and with temperatures that were estimated from injection current density ( Fig. 4b ). We may assume that in the temperature range of 10–60 K, the exciton binding energy does not change significantly, and the variation of InGaN bandgap is the dominant contributor to the emission peak energy over this temperature range. Also plotted in Fig. 4c is the measured variation of the EL excitonic peak energy with injected current density. Within the limits of experimental error the two curves follow each other very closely; the measured energy shift is marginally smaller than the theoretically predicted value. This suggests that there is no significant blue shift of the emission with injection, which is important in the context of single-photon emission. Figure 4: Single dot-in-nanowire p–n junction diode temperature. ( a ) Steady-state spatial temperature profile of a 600-nm-long nanowire of 30 nm diameter placed on a Si/SiO 2 platform for an injection current density of 283 A cm −2 . The scale bar denotes 30 nm. The silicon substrate is maintained at 10 K and the final nanowire temperature is ~59 K. ( b ) Calculated device temperature for different values of current density. The inset shows the transient response of the nanowire temperature for an injected current density of 283 A cm −2 . The transient response depends on the thermal resistance and capacitance of the system. ( c ) Emission energy shift as a function of the injected current density. The dots represent energy values calculated with the Varshni equation for equivalent temperatures corresponding to the current densities, obtained from the data shown in b . The error bars represent uncertainties in the Varshni fitting parameters. The squares represent measured variation of the exciton emission peak energy with injection current. Errors in the measurement arise from the resolution of the monochromator. Full size image Time-resolved PL We have investigated the temporal behaviour of the luminescence from the QD by time-resolved PL (TRPL) measurements at 10 K. The TRPL was measured using a single-photon detector following a high-resolution monochromator. The PL decay transient at the biexciton energy is shown in Fig. 5 . The measured data were analysed with the stretched exponential model: I = I o exp[−( t / τ ) β ], which yields values of the stretching parameter β =0.84±0.06 and a recombination lifetime of τ =711 ps. At the measurement temperature of 10 K, the latter represents the radiative lifetime of the biexciton emission, which is significantly lower than that measured in comparable In 0.25 Ga 0.75 N quantum wells [46] . This could be attributed to a relatively strong three-dimensional confinement that leads to a strong electron-hole overlap in the QD. The short radiative lifetime suggests the suppression of polarization field in the dot-in-nanowire heterostructure, as previously indicated by the invariance of the peak energy with excitation. It may also be noted that the QD biexciton decay lifetime measured here is significantly smaller than decay times reported for other nitride QD-based single-photon emitters [6] , [12] . The QD-nanowire diode is therefore promising as a single-photon source operating at high frequencies. 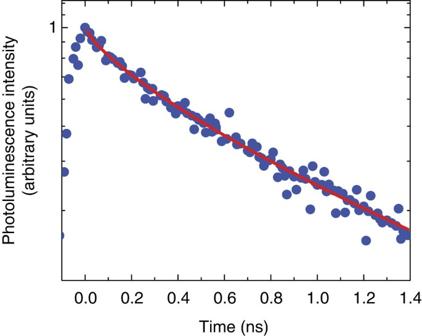Figure 5: Temporal variation of luminescence intensity from a single In0.25Ga0.75N dot-in-nanowire measured at the biexciton energy. The luminescence is detected at 10 K, by a single-photon avalanche photodiode with a response time of 40 ps. The solid curve indicates values calculated with the stretched exponential model. The fitting yields lifetimeτ=711 ps andβ=0.84±0.06. The adjustedR2value for the fit is 0.96. Figure 5: Temporal variation of luminescence intensity from a single In 0.25 Ga 0.75 N dot-in-nanowire measured at the biexciton energy. The luminescence is detected at 10 K, by a single-photon avalanche photodiode with a response time of 40 ps. The solid curve indicates values calculated with the stretched exponential model. The fitting yields lifetime τ =711 ps and β =0.84±0.06. The adjusted R 2 value for the fit is 0.96. Full size image Photon correlation statistics For an ideal single-photon source, the second-order correlation function: g (2) ( τ )=< I ( t ) I ( t + τ )>/< I ( t )>< I ( t + τ )>, where τ is the time delay and I ( t ) is the electroluminescence intensity at time t , should be equal to zero at zero time delay. 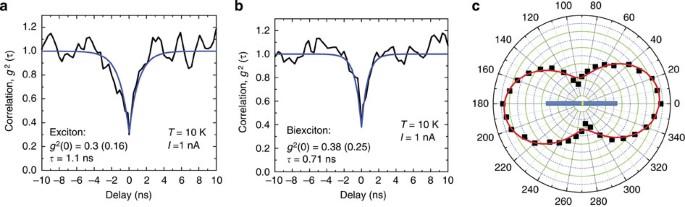Figure 6: Electrically injected single-photon emission from InGaN quantum dot-in-nanowire. Second-order correlation measured at 10 K with continuous electrical injection at (a) Exciton energy and (b) Biexciton energy. The solid lines are fits to the data as explained in the text. (c) Polar plot of electroluminescence intensity as a function of polarizer angle. The nanowire orientation is schematically superimposed. Figure 6a exhibit the second-order correlation measured in a standard Hanbury Brown and Twiss experiment for the exciton and biexciton resonances, respectively. The second-order correlation was measured under continuous excitation below saturation, at an injection current density of ~142 A cm −2 ( I =1 nA). The comparatively large separation between exciton and biexciton lines and narrow emission linewidths at 10 K allow us to spectrally filter and study each transition as a single-photon emitter. The dip in the correlation spectrum at zero time delay indicates anti-bunching in both exciton and biexciton complexes. We have analysed the correlation data for both peaks with the function: g (2) ( τ )=1− a × exp(− τ / b ) where (1− a ) and b are the g (2) (0) and recombination lifetime respectively. The solid lines represent the calculated values of g (2) ( τ ). The value of g (2) (0) for the exciton transition is 0.3, which corresponds to a 3-fold decrease in unwanted multi-photon emission events compared with attenuated coherent light sources. The anti-bunching dip is shallower in case of the biexciton emission, where g (2) (0)=0.38. This may be due to the faster recovery of g (2) ( τ ) of the biexciton with a shorter lifetime, compared with that of the exciton. The analysis gives exciton and biexciton emission lifetimes of 1.1 and 0.7 ns, respectively. The latter value is in excellent agreement with that obtained from the TRPL measurement. The finite value of the second-order correlation at zero time delay may be attributed to the finite time resolution of the measurement system and the background. To eliminate the effect of background counts, which could originate from stray light or merely dark counts, we apply a correction: g (2) (0)=1+( g (2) meas (0)−1)/ ρ 2 , where ρ is the ratio of signal-to-total counts, including dark counts [47] . The g (2) (0) values derived after background correction for the exciton and biexciton emission are 0.16 and 0.25, respectively. Figure 6: Electrically injected single-photon emission from InGaN quantum dot-in-nanowire. Second-order correlation measured at 10 K with continuous electrical injection at ( a ) Exciton energy and ( b ) Biexciton energy. The solid lines are fits to the data as explained in the text. ( c ) Polar plot of electroluminescence intensity as a function of polarizer angle. The nanowire orientation is schematically superimposed. Full size image Output polarization The polarization of the emitted single photons was also investigated by placing a linear polarizer in front of the monochromator. The measured intensity of the single dot biexciton emission as a function of the angle of the polarizer from the c axis of the nanowire is shown in the polar plot of Fig. 6c . The solid line indicates the fit of the experimental data to the function: I ( θ ) =a+b cos 2 ( θ–θ 0 ) where a and ( a + b ) are minimum and maximum values of the PL intensity, respectively, θ is the polarizer angle and θ 0 is the angle of polarization. The QD emission is linearly polarized with a degree of polarization, ρ =( I || − )/( I || + ) of ~70% along the c axis of the nanowire, where I || ( ) denotes the light intensity parallel (perpendicular) to the c axis of the nanowire. Strong linear polarization along the nanowire is attributed to the large dielectric constant contrast between the nanowire and the surrounding air, attenuating the electric field amplitude in the direction perpendicular to the nanowire [48] . It should be noted that the red shift in the QD emission due to increase of temperature associated with Joule heating is smaller than the value theoretically predicted by the Varshni equation. We attribute this difference to a small blue shift (<2 meV) that is likely to arise from the screening of the very small polarization field with excitation. As a consequence of the two competing effects, we observe that the excitonic emission remains almost invariant with injection. Typically, nitride-based quantum wells and self-organized QDs show blue shifts of the order of tens of meVs due to screening of the piezoelectric field and band filling of localized states [49] , [50] . The negligibly small blue shift in our device indicates that both these effects are greatly suppressed due to the dot-in-nanowire geometry. Pseudomorphic strain in InGaN/GaN and GaN/AlGaN nanowires has been known to relax efficiently at the sidewalls during growth [37] , [51] , [52] . Consequently, the piezoelectric field in such dot-in-nanowire heterostructures is significantly lower than that in quantum wells or self-organized QDs. Additionally, band filling effects induced by compositional inhomogeneities and alloy disorders, which lead to excitation dependent energy shifts, are also absent in this device. At 10 K, the biexciton decay time τ = τ rad =0.71 ns. The biexciton lifetime derived from analysis of the second-order correlation data is also 0.7 ns. The second-order correlation was measured at an injection current density of 142 A cm −2 , for which we estimate the actual device temperature to be ~25 K due to Joule heating. The close agreement between the two lifetime values indicates that the electrically injected carriers do not encounter recombination through non-radiative channels and both lifetime values correspond almost exclusively to radiative recombination. From temperature-dependent lifetime measurements performed on similar dot-in-nanowire ensemble samples, we have observed that the radiative lifetime is nearly constant with temperature. Hence, it can be assumed that the biexciton decay rate in our single dot device would be ~0.7 ns at higher temperatures. The relatively small radiative decay time is a remarkable advantage of the dot-in-nanowire geometry as it potentially allows for large repetition rates in single-photon emitters. Finally, the nanowires were grown on (111) Si and the single nanowire junction devices were fabricated on (001) Si, which make the single-photon sources reported here very attractive from the standpoint of compatibility and integration with silicon technology. However, operation of the device at higher temperatures will require engineering of the dot heterostructure to allow for better carrier confinement in the QD. Further optimization of the ohmic contact technology will be important to reduce the series resistance of the device. Due to growth-related inhomogeneities in the InGaN disk in the nanowires, the characteristics varied by a small degree from device to device. The results presented here represent the best ones measured. Epitaxial growth of nanowires on silicon The InGaN/GaN dot-in-nanowire heterostructure, shown schematically, was grown on (111) Si substrate by PA-MBE. After standard cleaning with solvents and removal of surface oxides with a dilute hydrofluoric acid solution, the substrate was annealed in the MBE chamber at 900 °C for 60 min before growth to remove any residual native oxide. Conventionally, the growth of GaN nanowires is initiated by depositing a few monolayers of Ga that act as a catalyst for subsequent growth of the nanowires. However, we found that under optimum growth conditions defect-free GaN nanowires can be grown on Si without the initial self-catalysis step. A striking difference in the nanowires grown by the two techniques lies in their diameters. It was observed that nanowires grown without the seed Ga deposition have an average diameters of ≤25 nm. Growth of the nanowire samples was carried out in a nitrogen-rich environment, while maintaining a constant N 2 flux of 1.0 s.c.c.m. The growth temperature was maintained at 800 °C and the Ga flux at 10 −7 Torr. Three hundred nanometre of Si-doped GaN ( n ~3 × 10 18 cm −3 ) was first grown, followed by the active region consisting of a 2-nm In 0.25 Ga 0.75 N QD at the centre of 30 nm of undoped GaN. During the growth of the QD, the substrate temperature was lowered to 535 °C and an in flux of 6 × 10 −8 Torr was used. Subsequently, 250 nm of Mg-doped p-type GaN ( p ~5 × 10 17 cm −3 ) was grown at 720 °C to allow for efficient Mg incorporation. The Mg flux was increased during the growth of the final 20 nm of p-GaN to achieve a better ohmic contact to a single nanowire. Lowering of the substrate temperature during the growth of p-GaN leads to an increase in the lateral growth rate and results in an increase in the nanowire diameter at the p-GaN end. TEM imaging Nanowires from the as-grown sample were mechanically removed from the substrate and ultrasonicated in isopropyl alcohol (IPA) for 20 min. Few drops of the nanowire IPA solution were then put on a carbon-coated TEM grid. After evaporation of the liquid, the nanowires on the grid were imaged using a JEOL 3011 high-resolution TEM. QD composition analysis STEM imaging and EDX measurements were performed on a single nanowire on a Cs-corrected JEOL 2100F TEM at an accelerating voltage of 200 kV. Before imaging and spectroscopy, the nanowires were dispersed on a holey carbon grid. A Hitachi SU8000 SEM with EDX capability was used to calibrate the Indium composition in InGaN nanowires, grown under identical conditions. Device fabrication The nanowires were dispersed on a (001) silicon wafer covered with 100 nm of thermal SiO 2 . Single nanowires were isolated by SEM imaging and Ti/Au ohmic contacts (5 nm/45 nm) with large contact pads were defined at the two ends of a single nanowire, ~600 nm in length, using electron beam lithography and electron beam evaporation techniques. The contacts were annealed in a N 2 ambient at 450 °C for 30 min and the devices were wire bonded onto chip carriers for measurements. Single dot spectroscopy and time-resolved PL Single QD spectroscopy was performed with a micro-PL measurement system in the far field in a confocal geometry. The sample was mounted on the cold finger of a continuous flow helium cryostat. Luminescence collected by an objective lens ( × 50) in the normal direction was analysed with a high-resolution monochromator with a spectral resolution of ~0.03 nm and detected with a photomultiplier tube using phase-sensitive lock-in amplification. For PL measurements, the same microscope objective was used to focus light from a frequency tripled Ti:sapphire laser ( λ =267 nm, repetition rate=80 MHz) on to the sample and to collect the luminescence from the InGaN/GaN QD. The photoexcitation spot size was ~5 μm and a pin hole was used to spatially resolve a single QD. For electroluminescence measurements, a continuous current is injected into the single nanowire device using a Keithley 6200 precision current source. For time-resolved PL measurements, the biexcitonic peak was filtered using a high-resolution monochromator and detected using a Picoquant single-photon avalanche photodiode with a response time of 40 ps. Second-order correlation measurements The second-order correlation of the exciton and biexciton was measured under continuous electrical excitation using a Hanbury Brown and Twiss measurement system. The exciton or biexciton luminescence was filtered from the QD emission and transmitted through a 50:50 beam splitter and on to two single-photon detectors, which provide the start and stop pulses to the counter. Temperature simulation The temperature of the nanowire was estimated by solving the Laplace equation for heat transfer using COMSOL Multiphysics software. The device is modelled as a uniform nanowire lying on 100 nm of thermal SiO 2 on the surface of a 500-μm silicon wafer, which is cooled to 10 K by the cold finger of the cryostat. The GaN region of the nanowire is the Joule heat source and the silicon wafer is effectively an infinite heat sink. The thermal oxide presents a thermal resistance between the nanowire and the heat sink. Heat loss due to convection may be ignored as the cryostat is evacuated before it is cooled down to 10 K. Radiation effects are also negligible as the temperature and area under consideration are small. Low temperature values of all material constants were considered. How to cite this article: Deshpande, S. et al . Electrically driven polarized single-photon emission from an InGaN quantum dot in a GaN nanowire. Nat. Commun. 4:1675 doi: 10.1038/ncomms2691 (2013).